Determining zebrafish dorsal organizer size by a negative feedback loop between canonical/non-canonical Wnts and Tlr4/NFκB In vertebrate embryos, the canonical Wnt ligand primes the formation of dorsal organizers that govern dorsal-ventral patterns by secreting BMP antagonists. In contrast, in Drosophila embryos, Toll-like receptor (Tlr)-mediated NFκB activation initiates dorsal-ventral patterning, wherein Wnt-mediated negative feedback regulation of Tlr/NFκB generates a BMP antagonist-secreting signalling centre to control the dorsal-ventral pattern. Although both Wnt and BMP antagonist are conserved among species, the involvement of Tlr/NFκB and feedback regulation in vertebrate organizer formation remains unclear. By imaging and genetic modification, we reveal that a negative feedback loop between canonical and non-canonical Wnts and Tlr4/NFκB determines the size of zebrafish organizer, and that Tlr/NFκB and Wnts switch initial cue and feedback mediator roles between Drosophila and zebrafish. Here, we show that canonical Wnt signalling stimulates the expression of the non-canonical Wnt5b ligand, activating the Tlr4 receptor to stimulate NFκB-mediated transcription of the Wnt antagonist frzb, restricting Wnt-dependent dorsal organizer formation. Animals display various body plans comprising various anatomical axes such as the dorsal-ventral (DV) and anterior-posterior (AP) axes. The establishment of body axes is one of the most fundamental events in the development of multicellular organisms. Since its discovery, the Spemann-Mangold organizer [1] , a group of cells that initiate DV axis formation in the amphibian embryo, has been intensively studied in a variety of model animals. It was found that organizer formation is induced by Wnt/β-catenin signaling. Canonical Wnt ligands, such as zebrafish Wnt8a and Xenopus Wnt11, activate β-catenin signaling, specifically in the dorsal embryonic region, thereby stimulating the formation of the dorsal organizer [2] , [3] , [4] , [5] , [6] . The dorsal organizer secretes the BMP antagonist Chordin into the ventral region; then, Chordin inhibits BMP-dependent ventral specification [7] , [8] , [9] . Thus, Wnt/β-catenin signaling initiates DV axis formation through Chordin/BMP in vertebrates. On the other hand, in Drosophila , the DV axis formation is initiated by Toll-like receptor (Tlr)/NFκB signaling [10] , [11] , [12] , [13] . Spätzle (Spz) ligands are proteolytically cleaved, specifically in the ventral-most region, which then activates the Tlr homolog (Toll). Activated Tlr stimulates the degradation of the IκB homolog, allowing nuclear translocation of the NFκB family of transcription factors and consequent transcriptional activation of genes for ventral specification [14] , [15] . Concurrently, NFκB also induces the expression of the Wnt family of extracellular protein WntD, functioning as an antagonist to attenuate Tlr/NFκB signaling [16] , [17] . This Wnt-mediated negative feedback regulation of Tlr/NFκB signaling is responsible for the precise size of the ventral embryonic region. Moreover, Tlr/NFκB signaling represses the BMP homolog (Dpp)-mediated dorsal specification by inducing the expression of the Chordin homolog (Sog) [18] , [19] . Thus, Tlr/NFκB signaling initiates Drosophila DV axis formation through the regulation of Wnt, Chordin, and BMP homologs. Taken together, Wnt, Chordin, and BMP are conserved mediators of DV axis formation in vertebrates and Drosophila . Since the Wnt/Chordin/BMP system is evolutionarily conserved and Drosophila Tlr/NFκB signaling initiates DV axis formation, it is expected that vertebrate Tlr/NFκB signaling might also be involved in DV axis formation. Overexpression of NFκB family genes reportedly inhibits dorsal formation in Xenopus laevis [20] , [21] . Other studies have shown that injection of Drosophila Spätzle and Tlr homolog into Xenopus embryos induced a secondary axis [22] , and that overexpression of IκB (inhibition of NFκB) blocked Xenopus dorsal formation [23] . While these findings indicate that Tlr/NFκB signaling may respectively function as a negative or positive regulator of dorsal formation, these overexpression studies remain controversial. Furthermore, although large-scale screening for isolating zebrafish mutants with dorsoventral patterning defects has been performed [24] , Tlr/NFκB signaling-related factors have not been isolated. Thus, the function and regulation of endogenous Tlr/NFκB signaling during vertebrate DV axis formation remain unclear. The negative feedback loop plays an important role in axis formation and size control. For example, a Sizzled-mediated BMP-Chordin feedback loop is required for correct DV patterning and embryonic size control [25] . Feedback regulation between Wnt and its secreted inhibitor Dkk1 contributes to size control of sensory organs [26] . The Wnt antagonist Sfrp1-mediated negative feedback regulation of Wnt/β-catenin signaling is essential for the development of a normal-sized heart muscle [27] . Because the dorsal organizer is the signaling center priming axis formation, organizer size should be properly controlled, raising the possibility that Wnt/β-catenin signaling, the organizer-inducer, may be restricted by negative feedback regulation. However, this mechanism is poorly understood. In this study, we examined the function and regulation of endogenous Tlr and NFκB during zebrafish DV axis formation, using a combination of in vivo reporter analysis, CRISPR/Cas9-mediated knockout, and morpholino knockdown. We show that during the initiation of dorsal organizer formation, Wnt/β-catenin signaling stimulates the activation of the NFκB homolog Rel through Toll-like receptor 4 (Tlr4), specifically in the dorsal embryonic tissue. Surprisingly, the non-canonical Wnt5 ligand mediates β-catenin-dependent Tlr4/Rel activation. Activated Rel then stimulates the transcription of a Wnt antagonist, frizzled-related protein ( frzb ), thereby restricting the Wnt/β-catenin-active area and dorsal organizer size. Thus, Wnt5-Tlr4/NFκB-mediated indirect negative feedback regulation of Wnt/β-catenin signaling determines the precise size of zebrafish dorsal organizer. NFκB activation in the dorsal region of zebrafish embryos To clarify the spatiotemporal pattern of NFκB activity, we generated a new NFκB reporter, NFκB-tkP:dGFP (Fig. 1a ). We confirmed that activation of NFκB stimulated NFκB-tkP:dGFP activity in human HEK293 cells (Supplementary Fig. 1a ) and then generated stable transgenic zebrafish lines carrying a single copy of NFκB-tkP:dGFP (Supplementary Fig. 1b ). NFκB-tkP:dGFP activity in transgenic fish was detected at 3.7 hours-post-fertilization (hpf) (Fig. 1b ), indicating that the reporter gene was zygotically activated. The reporter expression gradually accumulated to the dorsal margin of the blastoderm, which corresponds to the future dorsal organizer, from the dome stage (4.3 hpf), and completely localized in the dorsal region at the 50% epiboly stage (5.3 hpf) (Fig. 1b, c ). These results suggest that NFκB functions in dorsal organization. Fig. 1: Rel/NFκB negatively regulates dorsal organizer formation. a Schematic diagrams of NFκB-tkP:dGFP reporter. NFκB BS: consensus sequence of the NFκB-binding element. PolyA: SV40 polyadenylation sequence. b , c NFκB reporter is activated in the dorsal region of early zebrafish embryos. b Whole-mount in situ hybridization (WISH) for dGFP at the indicated stage in NFκB-tkP:dGFP-transgenic embryos. The dGFP -expressing dorsal regions are indicated with red arrowheads. Scale bar = 200 μm. c Double fluorescent in situ hybridization (FISH) for dGFP (green) and chordin (dorsal marker, magenta) in NFκB-tkP:dGFP-transgenic embryos. Animal views with dorsal to the right. Scale bar = 200 μm. d–f Inhibition of NFκB activity by iκbαb leads to expansion of organizer size and dorsal tissue. d WISH for dGFP in NFκB-tkP:dGFP-transgenic embryos, ( e ) dharma (organizer marker) and chordin in embryos injected with control (mKO2) or iκbαb mRNA at indicated stages. Animal views. Scale bar = 200 μm. Box plots of the angle of marker genes show first and third quartile, median is represented by a line, whiskers indicate the minimum and maximum. Each dot represents one embryo. P -values from unpaired two-tailed t -tests are indicated. f Phenotypes of larvae injected with control (mKO2) or iκbαb mRNA at 27 hpf. The strength of dorsalization was scored using the C1–5 classification scheme. Lateral views with anterior to the left. The loss of ventral tail fin (a typical dorsalization phenotype) is indicated with red arrowheads. Scale bar = 200 μm. g – i rel over-expression leads to reduction of organizer size and dorsal tissue. g WISH for dGFP in NFκB-tkP:dGFP-transgenic embryos, ( h ) dharma and chordin in embryos injected with control (mKO2) or rel mRNA at indicated stages. Scale bar =  200 μm. Box plots of the angle of marker genes show first and third quartile, median is represented by a line, whiskers indicate the minimum and maximum. Each dot represents one embryo. P -values from unpaired two-tailed t-tests are indicated. i Phenotypes of 27 hpf larvae injected with control (mKO2) or rel mRNA. The strength of ventralization was scored. Lateral views with anterior to the left. Scale bar = 200 μm. Source data are provided as a Source Data file. Full size image Rel/NFκB negatively regulates dorsal organizer formation To test whether NFκB is involved in dorsal organizer formation, we overexpressed the zebrafish IκB homolog iκbab to block NFκB activity in early zebrafish embryos (Fig. 1d ). Overexpression of iκbab induced expansion of the organizer area and dorsal tissue, marked by the expression of dharma and chordin , respectively [7] , [9] , [28] , [29] , [30] , in early embryos (Fig. 1e ), resulting in class 2–3 (C2–3) dorsalizations [31] , [32] , with a significant loss of ventral tail fin in larvae (Fig. 1f ). These results suggest that NFκB negatively regulates dorsal specification. Next, we investigated which NFκB regulates dorsal cell fate. In zebrafish, the NFκB family comprises five members: Rel (mammalian c-Rel homolog), Rela, Relb, NFκB1, and NFκB2 (Supplementary Fig. 2a ). We focused on Rel because it is the most homologous to Drosophila Dorsal, with high levels of rel transcripts being detected in early embryos (Supplementary Fig. 2a, b ). rel overexpression dramatically activated the NFκB reporter, narrowed the size of organizer and dorsal tissue, and reduced expression levels of the organizer marker dharma and the dorsal tissue marker chordin in early embryos (Fig. 1g, h and Supplementary Fig. 2c ). This induced the ventralized V1–4 phenotype in most larvae, characterized by the loss of dorsoanterior structures and expanded ventral tissues [32] (Fig. 1i ), which indicates that Rel may possibly inhibit the formation of dorsal organizer and dorsal tissue. To confirm this hypothesis, we used antisense morpholino (MO) to knockdown rel , blocking the translation of rel mRNA (Supplementary Fig. 2d ). Injection of rel MO dramatically reduced NFκB-tkP:dGFP activity (Fig. 2a ) and induced the expansion of dorsal tissues, marked by the expression of dharma and chordin , respectively (Fig. 2b and Supplementary Fig. 2e ), and the reduction of ventral tissues, marked by vent [33] (Fig. 2c ), resulting in class 2 (C2) dorsalization (Fig. 2d ). In addition, morpholino-resistant rel mRNA rescued rel MO-induced dorsal expansion (Supplementary Fig. 2f ). These results suggest that Rel restricts dorsal organizer formation and consequent dorsal specification. Although another NFκB gene, rela , is also expressed in early embryos (Supplementary Fig. 2b ), rela MO [34] did not affect the expression of dorsal marker genes (Fig. 2b and Supplementary Fig. 2g ) nor enhance rel MO-induced increase of dorsal gene expression (Supplementary Fig. 2g ). This suggests that Rel, but not Rela, is the main NFκB that acts in early zebrafish dorsal organizer formation. Fig. 2: Specific rel MO reveals that Rel restricts dorsal organizer formation. a Rel is a main NFκB acting in early zebrafish embryos. WISH for dGFP in NFκB-tkP:dGFP-transgenic embryos injected with control MO (ctrl MO) or rel MO at dome stage, animal view. Scale bar = 200 μm. b–d rel MO leads to expansion of organizer size and dorsal tissue in wild-type (WT) embryos whereas rela compensates the loss of rel in MZ rel embryos. WISH for ( b ) dharma , chordin , and ( c ) vent (ventral marker) in WT and maternal-zygotic rel mutants (MZ rel ) embryos injected with ctrl MO, rel MO or rela MO at 30% epiboly. Animal views with dorsal to the right. Scale bar = 200 μm. Box plots of the angle of marker genes show first and third quartile, median is represented by a line, whiskers indicate the minimum and maximum. Each dot represents one embryo. P -values from two-tailed one-way ANOVAs with Sidak correction are indicated. ns: not significant ( p > 0.05). d Representative pictures of 27 hpf WT and MZ rel larvae injected with ctrl MO, rel MO or rela MO. The strength of dorsalization was scored. The loss of ventral tail fin is indicated with red arrowheads. Lateral views with anterior to the left. Scale bar = 200 μm. e rela is upregulated in MZ rel but not rel morphants. qPCR analysis for expression of rela in MZ rel or rel morphants at sphere stage. Normalized values are shown as means ± SEM. n = 3, biologically independent samples. P -values from unpaired two-tailed t-tests are indicated. f Model of the mechanism of rela- mediated genetic compensation and the specific inhibition by rel MO. Source data are provided as a Source Data file. Full size image Upregulation of rela compensates the genetic loss of rel To confirm the role of rel , we generated a rel mutant by CRISPR/Cas9-mediated knockout, which has a frameshift in the Rel homology domain, leading to early termination of translation (Supplementary Fig. 2h ). We also confirmed that rel expression was dramatically decreased in the maternal-zygotic rel mutants (MZ rel ) (Supplementary Fig. 2i ). Unexpectedly, MZ rel embryos exhibited no gross morphological defects (Fig. 2d , top-right panel). Consistent with this, there were no significant differences in the expression of dorsal marker genes between wild-type (WT) and MZ rel embryos (Fig. 2b and Supplementary Fig. 2e ). A previous study showed that the lack of a mutant phenotype is due to the upregulation of either gene paralogs or genes with sequence homology [35] , [36] , [37] . We found that rela was significantly upregulated in MZ rel , but not rel morphants (Fig. 2e, f ). Moreover, injection of rela MO enhanced the expression of dorsal markers (Fig. 2b ) and induced dorsalized phenotypes in MZ rel embryos, but not in WT embryos (Fig. 2d, f ). These results indicate that the upregulation of rela compensates for the genetic loss of rel in mutants but not rel morphants (Fig. 2f ). Notably, MZ rel is rel MO-resistant, with no obvious defects after rel MO injection (Fig. 2b, d, f and Supplementary Fig. 2e ), indicating that MZ rel is a null mutant and that rel MO specifically inhibits the function of rel . Therefore, we used this specific morpholino to investigate the functions of Rel. Rel inhibits Wnt signaling through activating Frzb Given that Wnt/β-catenin initiates the formation of the dorsal organizer, we investigated whether Rel regulates Wnt/β-catenin signaling. Injection of rel MO resulted in a significant increase in axin2 and sp5l , the specific targets of Wnt/β-catenin activity [38] (Fig. 3a, b and Supplementary Fig. 3a ). Consistently, rel overexpression significantly decreased the expression of Wnt target genes (Fig. 3c, d ). However, rel MO did not affect the expression of Nodal ( ndr1 and ndr2 ) [39] and BMP signaling target genes ( foxi1 and bambia ) [40] , [41] , which are also involved in DV axis formation [42] , at the early stage of dorsal organizer induction (Supplementary Fig. 3b ). These results suggest that Rel selectively inhibits Wnt/β-catenin signaling during organizer formation. Fig. 3: Rel negatively regulates Wnt/β-catenin signaling. Wnt/β-catenin signaling is enhanced by rel knockdown ( a , b ) and decreased by rel overexpression ( c , d ) at the dome stage. WISH ( a , c ) and qPCR analysis ( b , d ) of axin2 and sp5l in dome-stage WT embryos injected with ctrl MO, rel MO, control (mKO2) or rel mRNA. In a and c , animal views are shown. Scale bar = 200 μm. In b and d , normalized values are shown as mean ± SEM. n = 3 biologically independent samples. P -values from unpaired two-tailed t -tests are indicated. Source data are provided as a Source Data file. Full size image Next, we investigated how Rel negatively regulated Wnt/β-catenin signaling. As Rel functions as a transcription factor with a transactivation domain, we hypothesized that Rel stimulates the expression of Wnt/β-catenin signaling inhibitors. Therefore, we examined the expression of Wnt antagonists in early zebrafish embryos [6] , [43] . Knockdown of rel significantly reduced the expression of the Wnt antagonist frzb in the dorsal margin but had no significant effect on the expression of other Wnt antagonists (Fig. 4a, b and Supplementary Fig. 3a, b ), whereas rel overexpression enhanced frzb expression (Supplementary Fig. 3c ). These outcomes suggest that Rel selectively activates Frzb expression. Consistent with a previous study [6] , we confirmed that frzb knockdown using MO induced the upregulation of the Wnt target gene axin2 and dorsal expansion phenotypes, whereas overexpression of frzb induced the opposite effects (Supplementary Fig. 4a–c ). Moreover, rel MO-induced Wnt/β-catenin activation and dorsal expansion were restored by co-injection with frzb mRNA (Fig. 4c, d ), suggesting that Rel inhibited Wnt/β-catenin signaling by inducing Frzb expression. It is worth noting that overexpression of sfrp1a also rescued rel MO-induced activation of Wnt signaling and dorsal expansion (Supplementary Fig. 4d, e ). This suggests that antagonizing Wnt ligand activity is important for size control of the dorsal organizer. Fig. 4: Rel directly activates a secreted Wnt antagonist Frzb to restrict Wnt/β-catenin-mediated dorsal organizer formation. a , b Rel positively regulates frzb expression. a qPCR analysis for expression of Wnt antagonists ( frzb , sfrp1a , dkk1b and notum1a ) in dome stage embryos injected with ctrl MO or rel MO. Normalized values are shown as means ± SEM. n = 3, biologically independent samples. P -values from unpaired two-tailed t-tests are indicated. b WISH for frzb in dome stage embryos injected with ctrl MO or rel MO, animal view. c , d Rel inhibits Wnt/β-catenin signaling through Frzb. WISH for ( c ) Wnt targets axin2 and sp5l ; ( d ) dharma and chordin in embryos injected with ctrl MO, rel MO or rel MO with frzb mRNA at indicated stage, animal view. Box plots of the angle of marker genes show first and third quartile, median is represented by a line, whiskers indicate the minimum and maximum. Each dot represents one embryo. P -values from two-tailed one-way ANOVAs with Sidak correction are indicated. e , f Rel activates promoter of frzb . e Top panel shows the schematic diagram of the upstream region of zebrafish frzb gene. The NFκB-binding element possessing the strongest potential to bind to Rel homodimer is marked with red “pin” while others are marked by black “pins”. Gray and blue boxes indicate Exons and UTRs, respectively. Bottom panel shows the schematic diagrams of the reporter constructs, frzb:luc and frzb:luc MT. f FISH for luciferase (magenta) and gfp (green) in dome-stage embryos injected with pDha-GFP and frzb:luc or frzb:luc MT, with MOs as indicated, animal view. Scale bar = 200 μm. Source data are provided as a Source Data file. Full size image We also discovered three elements that possess binding potential to Rel 2 kb upstream of the zebrafish frzb gene (Fig. 4e ), using the NFκB-binding elements search tool [44] . Among these, the element that was nearest to frzb gene (−246–236 bp) had the strongest binding potential to Rel (Fig. 4e ). To examine whether Rel directly activates frzb transcription, we generated a frzb :luc reporter in which a 500 bp promoter sequence, including the potential Rel-binding element, was fused with the luciferase gene and the Rel-binding element-deleted mutant (MT) reporter frzb :luc MT (Fig. 4e ). Embryos injected with frzb :luc, but not with frzb :luc MT, expressed luciferase mRNA in the dorsal organizer region, which was confirmed by co-injection with the organizer reporter pDharma-GFP [45] (Fig. 4f ). Knockdown of rel decreased the activity of frzb :luc reporter, whereas overexpression of rel activated it (Fig. 4f and Supplementary Fig. 3d ). These results suggest that Rel directly activated frzb promoter through the Rel-binding element. Tlr4 activates NFκB to stimulate frzb expression Next, we investigated NFκB activation. Because Tlr/NFκB signaling determines Drosophila DV axis, we investigated whether Tlr mediates NFκB activation in early zebrafish embryos. We focused on Tlr4 because it is highly expressed among Tlrs in early zebrafish embryos [46] . We confirmed that tlr4 was expressed in early zebrafish embryos (Supplementary Fig. 5a ). Similar to rel knockdown, injection of a dominant-negative mutant of Tlr4 (Tlr4 DN) [47] or treatment with the Tlr4-specific inhibitor TAK-242 [48] , [49] induced a reduction in NFκB reporter activity and frzb expression and the upregulation of the Wnt target gene axin2 , the dorsal organizer gene dharma , and the dorsal marker chordin (Fig. 5a, b and Supplementary Fig. 5b–d ) and consequent dorsalized phenotype (Fig. 5c and Supplementary Fig. 5e ). Furthermore, forced activation of Tlr4 by injection of lipopolysaccharide (LPS), which is an exogenous Tlr4 ligand derived from the cell wall of gram-negative bacteria [50] , induced a ventralized phenotype at 27 hpf (Fig. 5d ). LPS significantly activated the NFκB reporter and enhanced frzb expression, which was restored by either Tlr4 DN injection or TAK-242 treatment (Fig. 5e and Supplementary Fig. 5f ). Moreover, LPS injection decreased the expression of the Wnt target gene axin2 and the dorsal marker genes dharma and chordin (Fig. 5f and Supplementary Fig. 5g ). These results suggest that Tlr4 activates NFκB to stimulate frzb -mediated restriction of dorsal organizer formation. Fig. 5: Tlr4 activates NFκB to stimulate frzb -mediated restriction of dorsal organizer formation. a – c Inhibition of Tlr4 reduces frzb expression and enhances Wnt/β-catenin signaling and dorsal organizer formation. Embryos were injected with mKO2 (control) or Tlr4 DN mRNA. WISH for ( a ) dGFP in NFκB-tkP:dGFP-transgenic; frzb and axin2 in WT, ( b ) dharma and chordin in WT embryos at the indicated stage. Animal views. Box plots of the angle of marker genes show first and third quartile, median is represented by a line, whiskers indicate the minimum and maximum. Each dot represents one embryo. P -values from unpaired two-tailed t-tests are indicated. c Representative pictures of 27 hpf larvae, lateral views with anterior to the left. The strength of dorsalization was scored. d – f Forced activation of Tlr4 by injection of lipopolysaccharide (LPS) activates NFκB signaling and inhibits dorsal organizer formation. d Phenotypes of 27 hpf larvae injected with LPS, uninjected as control. The strength of ventralization was scored. Lateral views with anterior to the left. e Embryos were injected with LPS and treated with DMSO or TAK-242 or co-injected with Tlr4 DN, uninjected as control. DMSO and TAK-242 were treated from 3 hpf to dome stage. WISH for dGFP in NFκB-tkP:dGFP-transgenic; frzb in WT embryos at dome stage. f WISH for axin2 , dharma and chordin in embryos injected with LPS, uninjected as control. Animal views. Scale bar = 200 μm. Source data are provided as a Source Data file. Full size image β-catenin stimulates Wnt5-mediated Tlr4/NFκB activation Since Wnt/β-catenin signaling and NFκB are activated in the dorsal region, it is possible that Wnt/β-catenin also regulates NFκB signaling. Interestingly, forced activation of Wnt/β-catenin signaling by a constitutively active β-catenin mutant (β-cat CA) dramatically enhanced NFκB reporter activity and frzb expression, which was reversed by co-injection with Tlr4 DN (Fig. 6a ). In contrast, knockdown of the β-catenin homolog ctnnb2 by translation-blocking MO [51] decreased both NFκB reporter activity and frzb expression (Fig. 6b ). These results suggest that Wnt/β-catenin signaling activates NFκB through Tlr4. Consistent with this, the Wnt/β-catenin reporter OTM:d2EGFP [52] was initially activated at 3.7 hpf, which is earlier than the NFκB reporter and NFκB target gene frzb (Fig. 6c ). Thus, Wnt/β-catenin and Tlr4/NFκB form an indirect negative feedback loop. Fig. 6: β-catenin stimulates Wnt5b-mediated Tlr4/NFκB activation. a , b β-catenin activates NFκB via Tlr4. a Embryos were injected with control (mKO2) or constitutively active β-catenin mutant (β-cat CA) mRNA, with or without Tlr4 DN mRNA. b Embryos were injected with control or ctnnb2 (zebrafish β-catenin) MO. WISH for dGFP in NFκB-tkP:dGFP-transgenic; frzb in WT embryos at the dome stage, animal view. Scale bar = 200 μm. c NFκB is activated following Wnt/β-catenin activation in the developing dorsal organizer. WISH for dGFP in OTM:d2EGFP and NFκB-tkP:dGFP-transgenic embryos and frzb in WT embryos at the indicated stage. The dGFP -expressing and frzb -expressing dorsal regions are indicated by red arrowheads. Scale bar = 200 μm. d β-catenin activates wnt5b expression in early embryos. Embryos were injected with control (mKO2) or constitutively active β-catenin mutant (β-catCA) mRNA. WISH for wnt5a and wnt5b at the sphere stage, animal view. Scale bar = 200 μm. e , f Wnt/β-catenin signaling activates NFκB via Wnt5b. e Embryos were injected with ctrl or wnt5b MO. f Embryos were injected with control (mKO2) or constitutively active β-catenin mutant (β-cat CA) mRNA, with or without wnt5b MO. WISH for dGFP in NFκB-tkP:dGFP-transgenic embryos at the dome stage, animal view. Scale bar = 200 μm. g , h Wnt5b activates frzb expression through Tlr4/Rel. g Embryos were injected with control (mKO2) or wnt5b mRNA, and co-injected with Tlr4 DN mRNA or rel MO. WISH for dGFP in NFκB-tkP:dGFP-transgenic, frzb in WT embryos at the dome stage, animal view. Scale bar = 200 μm. h WISH for dharma in WT embryos injected with control (mKO2) or wnt5b mRNA at 30% epiboly stage. Scale bar = 200 μm. Box plots of the angle of marker gene show first and third quartile, median is represented by a line, whiskers indicate the minimum and maximum. Each dot represents one embryo. P -values for unpaired two-tailed t-tests are indicated. Source data are provided as a Source Data file. Full size image As tlr4 genes are ubiquitously expressed, we hypothesized that Wnt/β-catenin may stimulate the expression of a Tlr4 ligand in the dorsal region. A recent study showed that the non-canonical Wnt ligand Wnt5 is a Tlr4 ligand in human myeloid cell cultures [53] . Moreover, similar to Tlr4/NFκB, Wnt5 negatively regulates dorsal formation by blocking Wnt/β-catenin signaling [54] , [55] , [56] , [57] . In particular, the endogenous wnt5b gene negatively regulates zebrafish dorsal organizer formation. Therefore, we tested whether β-catenin activates Tlr4/NFκB through Wnt5b. We found that wnt5b was specifically expressed in the dorsal region (Supplementary Fig. 6a ) and significantly activated after β-cat CA injection, whereas the expression of another Wnt5 gene, wnt5a , was not detected (Fig. 6d ), indicating that wnt5b is a β-catenin target gene in early zebrafish embryos. Furthermore, knockdown of Wnt5b using wnt5b translation-blocking MO [58] decreased the NFκB activity significantly (Fig. 6e ) and reversed β-cat CA-induced NFκB activation (Fig. 6f ), suggesting that β-catenin activates Tlr/NFκB signaling through Wnt5b. Consistent with this idea, overexpression of wnt5b mRNA significantly enhanced NFκB reporter and frzb expression which were restored by either Tlr4 DN or rel MO injection (Fig. 6g and Supplementary Fig. 6b ). In addition, Wnt5b overexpression also inhibited dorsal organizer formation (Fig. 6h ). Taken together, Wnt/β-catenin signaling appears to activate Tlr4/NFκB through the non-canonical Wnt ligand, Wnt5b. In this study, we demonstrate that the Tlr4/NFκB-mediated negative feedback regulation of Wnt/β-catenin signaling determines the precise size of the zebrafish dorsal organizer. In early zebrafish embryos, Wnt/β-catenin signaling stimulates the transcription of the non-canonical Wnt5b ligand, which activates the NFκB protein Rel through Tlr4 in the dorsal region. Rel stimulates the transcription of the Wnt antagonist frzb , thereby restricting the Wnt/β-catenin-active area and dorsal organizer size. Similar to Drosophila , zebrafish determine their embryonic DV axis through negative feedback regulation between Tlr/NFκB and Wnt. Interestingly, the roles of these factors appear to be switched between these two species. Tlr/NFκB acts as the initial cue of DV axis formation in Drosophila and as a feedback mediator in zebrafish, whereas Wnt functions as the initial cue in zebrafish and as a feedback mediator in Drosophila (Fig. 7 ). Fig. 7: Negative feedback loop between canonical/non-canonical Wnts and Tlr4/NFκB determines the precise size of zebrafish dorsal organizer. Model of the role of Tlr/NFκB signaling in the initiation of embryonic DV axis formation. In Drosophila , Wnt-mediated negative feedback regulation of Toll/NFκB signaling determines the embryonic DV pattern. In zebrafish, negative feedback regulation between canonical Wnt (caWnt), non-canonical Wnt (Wnt5b), and Tlr4/NFκB generates the precise size of the dorsal organizer and the consequent DV pattern. Full size image To precisely generate embryonic tissue of specific size, morphogen signaling is adjusted for correct distribution. Negative feedback regulation measures tissue size and buffer variability. For example, the sizes of sensory organs and heart muscles are correctly determined by negative feedback regulation between Wnt and its secreted antagonists Dkk1 and Sfrp [26] , [27] . The dorsal organizer is formed by Wnt and expresses secreted Wnt antagonists, including Frzb [6] , [59] , which raises the possibility that negative feedback regulation between Wnt and antagonists may be involved in organizer size control. However, such feedback regulation remains unreported, and the mechanisms by which Frzb expression is controlled in organizer remain unclear. In this study, we show that a previously unidentified “indirect” negative feedback loop, consisting of Wnt, Tlr4/NFκB, and Frzb, restricts the size of the dorsal organizer. Interestingly, Wnt indirectly activates Frzb through Tlr4/NFκB, whereas the well-studied Wnt negative feedback regulator Dkk1 is a direct Wnt target gene [60] , [61] . The significance of “indirect” feedback lies in the fact that while it is known that a “direct” autoregulatory feedback loop can shorten the response time of a network, indirect feedback via intermediate genes can generate time delay [62] , [63] , [64] . If Wnt signaling is inhibited through direct negative feedback during organizer induction, Wnt signaling would be immediately shut off and would not be able to form an organizer of an adequate size. Indirect negative feedback delays the timing of Wnt inhibition, which may ensure an adequate duration for Wnt diffusion and consequent formation of a properly sized organizer (Supplementary Fig. 7 ). Since the discovery of Tlr/NFκB (Toll/Dorsal) signaling as an initiator of Drosophila DV axis formation [10] , [11] , [12] , [13] , the involvement of Tlr/NFκB signaling in vertebrate DV axis formation has been expected. However, no related factors were found in large-scale screening for isolating zebrafish mutants with dorsoventral patterning defects [24] . Furthermore, previous Xenopus studies showed that dorsal formation can be blocked by overexpression not only of NFκB [20] , [21] but also of IκB [23] , indicating that these overexpression analyses are controversial and potentially insufficient to prove the contribution of these factors to axis formation. Moreover, while mutant mice with disrupted key components of the Tlr/NFκB pathway demonstrated immune deficiency, no significant defects in body axis formation were observed [65] , [66] , [67] , [68] . Genetic compensation can reportedly buffer the organism against gene loss that would otherwise be deleterious to survival, whereas morpholino-mediated knockdown blocked the target gene immediately and induced no genetic compensation [35] , [36] , [37] , suggesting that both knockout and knockdown analyses are required to clarify endogenous gene function. Here, we show that genetic compensation masks the roles of Rel, a member of the NFκB family, in early zebrafish embryos, and we clarify the hidden roles of Rel during DV axis formation by the combinatorial analyses. rel knockout mutants generated using CRISPR/Cas9 have no significant embryonic defects, whereas MO-mediated knockdown and in vivo imaging analyses revealed the involvement of rel in dorsal organizer formation. The upregulation of another rel homolog, rela , compensates for the loss of rel in the mutant. Thus, by taking advantage of knockdown, knockout, and imaging, we succeeded in discovering the previously unknown function and regulation of NFκB in vertebrate axis formation. Our finding is consistent with the previous Xenopus studies showing that overexpression of Xrel3 or XrelA (homolog of zebrafish Rel or Rela, respectively) inhibited the dorsal formation and the dorsal marker gene expression [20] , [21] , which indicates that endogenous Xrel3 and XrelA may play roles similar to zebrafish Rel and Rela in Xenopus organizer formation. The present study shows that Tlr/NFκB activates the transcription of Frzb to inhibit canonical Wnt ligands. Notably, the frzb promoter region of other vertebrates contains several potential NFκB-binding elements, including in Xenopus , chicken, and mouse (Supplementary Fig. 3e ), which also generate organizer structures through Wnt/β-catenin signaling [1] , [69] , [70] , [71] , [72] . This suggests the potentially conserved roles of the Tlr-NFκB-Frzb-Wnt axis in organizer formation across widely different taxa. Interestingly, whereas dorsally activated Wnt/β-catenin signaling in zebrafish initiates DV axis formation and negatively regulates itself through Tlr/NFκB-mediated indirect induction of the Wnt antagonist Frzb, ventrally activated Tlr/NFκB primes DV patterning and negatively control its activity through direct induction of WntD expression in Drosophila (Fig. 7 ). This ventral Tlr/NFκB-driven DV patterning is observed not only in Drosophila but also in other insects, such as Tribolium and Gryllus [73] , [74] , [75] . Thus, the roles of Tlr/NFκB have changed in the course of evolution. This change seems to be associated with the appearance of Wnt/β-catenin signaling-mediated organizer formation and NFκB-mediated Wnt antagonist (Frzb) induction. In fact, Wnt/β-catenin signaling is required for the formation of the Chordin-secreting organizer in vertebrates, amphioxus (a cephalochordate) [76] , and the region functionally equivalent to the organizer in sea urchins (echinoderms) [77] , [78] , whereas Wnt/β-catenin activity is not involved in the initial induction of the signaling centre organizing DV patterning in insects including Drosophila . Furthermore, the Sfrp3/4 subfamily of Wnt antagonist genes, to which frzb (also called Sfrp3) belongs [79] , is found in the genome of vertebrates, cephalochordates, and echinoderms, which possess the organizer or related structures [76] , [78] , but not in that of insects and nematodes, which do not [80] . It may be concluded that the evolutionary acquisition of organizer formation mediated by Wnt and its antagonist (Frzb) enabled vertebrates, cephalochordates, and echinoderms to change the roles of Tlr/NFκB from ‘initiator’ to ‘mediator between Wnt and Frzb’ in DV patterning. We also demonstrate that the Toll-like receptor Tlr4 mediates Rel activation downstream of Wnt/β-catenin signaling during organizer formation using a specific inhibitor and a dominant-negative mutant. Although Tlr4 was first identified as a receptor of LPS derived from gram-negative bacteria [50] , [67] , many endogenous Tlr4 ligands, including hyaluronan and fibronectin, have also been identified [81] , [82] . A recent study using primary cell cultures and in vitro binding experiments also showed that Wnt5 can directly bind to Tlr4 to stimulate NFκB activation [53] . Previous zebrafish studies have shown that zygotic expression of wnt5b is induced during the organizer formation stage [6] and that maternal-zygotic wnt5b mutants exhibit organizer size expansion [57] like Tlr4-inhibited embryos and rel morphants. The Wnt5 subclass is called a non-canonical Wnt ligand and negatively regulates β-catenin signaling-mediated dorsal formation by activating the Ca 2+ pathway [54] , [55] , [56] , [57] . However, the mechanisms controlling wnt5b expression in early zebrafish embryos and the role of Wnt5 as a Tlr4 ligand in vivo remain unclear. Here, we demonstrate that Wnt/β-catenin signaling stimulates wnt5b expression in developing organizer and that Wnt5b acts as a potential Tlr4 ligand to block Wnt/β-catenin signaling. Thus, our study revealed previously unidentified interactions between the canonical and non-canonical Wnt signaling pathways. Although several transgenic NFκB reporter lines have been generated in zebrafish and mice, the activation of NFκB was not detected in early embryos around the initial stage of DV axis formation [83] , [84] , [85] . In this study, we successfully detected spatiotemporal activation of NFκB in early embryos using a transgenic zebrafish reporter. Interestingly, NFκB activation was detected as a “salt and pepper pattern” from 3.7 hpf and then restricted to the dorsal region from 4.3 hpf (Fig. 1b ). The significance of the earliest salt-and-pepper pattern is still unclear. Although germ cells also showed a dotty pattern in early zebrafish embryos [86] , [87] , they did not express NFκB reporter (Supplementary Fig. 1d ), indicating that NFκB is activated in other cells. It is important to investigate this NFκB activation to fully understand the roles of endogenous NFκB during vertebrate embryogenesis. Bacterial infections during pregnancy have been linked to various negative pregnancy outcomes, including spontaneous abortion, premature birth, stillbirth, intrauterine growth restriction, and fetal neurological defects in humans [88] , [89] , [90] . Tlr4 is a well-known sensor that recognizes the presence of bacterial infection [91] , [92] . A previous study reported that early mouse embryos express Tlr4 [93] , [94] , and maternal LPS elevated by bacterial infection negatively affects mouse fetal development and induces intra-uterine fetal death [95] . However, the mechanisms by which bacterial infection affects embryonic development are not fully understood. The current consensus is that inflammatory cytokines and chemokines, which are small immunological proteins, likely play a central role in infection-associated preterm birth and fetal injury [90] , [95] . In our study, we found that LPS severely interrupts zebrafish embryonic axis formation through Tlr4/NFκB signaling, which provides a previously undescribed mechanism of bacteria-induced defects in embryogenesis. We expect that our study using zebrafish as a model can deepen insights into the mechanisms by which infection influences early embryonic development. Ethical approval All experimental animal care was performed in accordance with the institutional and national guidelines and regulations. The study protocol was approved by the Institutional Animal Care and Use Committee of Osaka University (RIMD Permit# R02-04). The study was conducted according to the ARRIVE guidelines. Zebrafish maintenance Zebrafish Wild-type strain (AB), Tg(OTM:d2EGFP) [52] , Tg(NFκB-tkP:dGFP), and rel mutant were raised and maintained under standard conditions. Tg(NFκB-tkP:dGFP) and rel mutant were generated in this study. Assays were conducted in zebrafish embryos and larvae at 3–27 hpf. At these developmental stages, sex is not yet determined. All experimental animal care was performed in accordance with the institutional and national guidelines and regulations. Reporter plasmid construction To produce the reporter plasmid NFκB-tkP:dGFP, the Tcf/Lef-binding sequence and the minimal promoter of the OTM:d2EGFP (Tcf/Lef-miniP:dGFP) plasmid [52] was replaced with six copies of consensus NFκB binding sites (CTCGAGCGGAAAGTCCCACGGAAAGTCCCACGGAAAGTCCCACGGAAAGTCCCACGGAAAGTCCCACGGAAAGTCCCA) [96] and a thymidine kinase (tk) minimal promoter (tkP: CCCGCCCAGCGTCTTGTCATTGGCGAATTCGAACACGCAGATGCAGTCGGGGCGGCGCGGTCCCAGGTCCACTTCGCATATTAAGGTGACGCGTGTGGCCTCGAACACCGAGCGACCCTGCAG). The NFκB-binding element search tool ( http://thebrain.bwh.harvard.edu/nfkb/ ) predicted that all NFκB family members could bind to these consensus NFκB binding sites on the reporter gene. Generation of transgenic and mutant zebrafish For NFκB-tkP:dGFP transgenic zebrafish, 50 pg reporter plasmid DNA with 25 pg Tol2 transposase mRNA was injected into one-cell-stage wild-type zebrafish (AB) embryos. Transgenic fish that strongly expressed dGFP were outcrossed with wild-type fish to produce a transgenic line carrying a single transgene, Tg (NFκB-tkP:dGFP). This line was maintained as homozygous transgenic fish. For CRISPR/Cas9-mediated generation of rel knockout mutant zebrafish, gRNA design and in vitro transcription of Cas9 RNA were performed according to previously reported protocols [97] . Cas9 mRNA and gRNA were synthesized in vitro and co-injected into one-cell-stage wild-type zebrafish (AB) embryos. The sequence of the selected CRISPR target site was 5′-CGTTCTGCGGGCAGCATACC AGG −3′ (bold lettering indicates the PAM motif). Adult F0 fish were outcrossed with AB WT fish, and DNA was extracted from F1 progeny. Mutations were identified through direct sequencing of the PCR amplicon comprising the CRISPR target region. Plasmids The zebrafish iκbαb , rel , frzb , sfrp1a , and wnt5b coding sequences were amplified using a zebrafish cDNA library. The mKO2 cDNA was purchased from MBL (Tokyo, Japan). rel 5′ untranslated regions were annealed by DNA oligos, and cDNA for mKO2 was PCR-amplified. These two DNA fragments were cloned into the multi-cloning site of the pCS2p+ vector using the In-Fusion® HD Cloning Kit (Takara, Kusatsu, Japan). The dominant negative form of Tlr4 was PCR-amplified from mouse Tlr4 (Addgene #13085) with deletion of the TIR domain [47] . The N-terminus truncated mouse β-catenin (β-cat CA) has been described previously [98] . To prepare frzb -luciferase plasmid, the frzb gene upstream region (−500-1), including a putative NFκB binding site (TGTAGTTTCC), was amplified from a zebrafish genomic library and inserted upstream of the firefly luciferase gene in the pGL4 vector (Promega, Madison, WI, USA). A mutant reporter, in which a putative NFκB-binding site was deleted, was generated using the QuikChange Site-Directed Mutagenesis Kit (#210518; Agilent, Santa Clara, CA, USA). The pDha-1420GFP plasmid has been previously described [45] . Injection of mRNA, plasmid, morpholino, and LPS Capped mRNA was synthesized using the SP6 mMessage mMachine Kit (Ambion, Austin, TX, USA) and purified using Micro Bio-Spin columns (Bio-Rad, Hercules, CA, USA). We injected synthesized mRNA (50 pg of iκbαb , 10 pg of rel , 500 pg of frzb , 500 pg of sfrp1a , 2 ng of Tlr4 DN, 20 pg of β-cat CA, and 120 pg of wnt5b ) at the one-cell stage of zebrafish embryos. Antisense oligo MOs (Gene Tools, Philomath, OR, USA) were injected into one-cell-stage embryos. Translation-blocking morpholinos used were rel MO (5 ng), rela MO (3 ng) [34] , frzb MO (10 ng) [6] , ctnnb2 MO (10 ng) [51] , wnt5b MO (8 ng) [58] and standard control (3–10 ng). 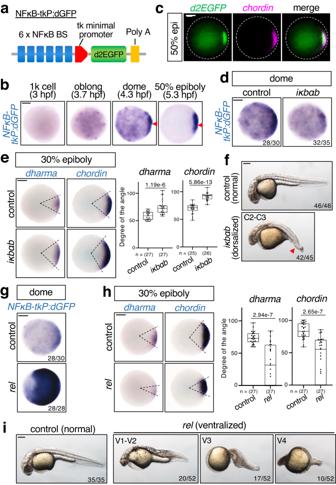Fig. 1: Rel/NFκB negatively regulates dorsal organizer formation. aSchematic diagrams of NFκB-tkP:dGFP reporter. NFκB BS: consensus sequence of the NFκB-binding element. PolyA: SV40 polyadenylation sequence.b,cNFκB reporter is activated in the dorsal region of early zebrafish embryos.bWhole-mount in situ hybridization (WISH) fordGFPat the indicated stage in NFκB-tkP:dGFP-transgenic embryos. ThedGFP-expressing dorsal regions are indicated with red arrowheads. Scale bar = 200 μm.cDouble fluorescent in situ hybridization (FISH) fordGFP(green) andchordin(dorsal marker, magenta) in NFκB-tkP:dGFP-transgenic embryos. Animal views with dorsal to the right. Scale bar = 200 μm.d–fInhibition of NFκB activity byiκbαbleads to expansion of organizer size and dorsal tissue.dWISH fordGFPin NFκB-tkP:dGFP-transgenic embryos, (e)dharma(organizer marker) andchordinin embryos injected with control (mKO2) oriκbαbmRNA at indicated stages. Animal views. Scale bar = 200 μm. Box plots of the angle of marker genes show first and third quartile, median is represented by a line, whiskers indicate the minimum and maximum. Each dot represents one embryo.P-values from unpaired two-tailedt-tests are indicated.fPhenotypes of larvae injected with control (mKO2) oriκbαbmRNA at 27 hpf. The strength of dorsalization was scored using the C1–5 classification scheme. Lateral views with anterior to the left. The loss of ventral tail fin (a typical dorsalization phenotype) is indicated with red arrowheads. Scale bar = 200 μm.g–irelover-expression leads to reduction of organizer size and dorsal tissue.gWISH fordGFPin NFκB-tkP:dGFP-transgenic embryos, (h)dharmaandchordinin embryos injected with control (mKO2) orrelmRNA at indicated stages. Scale bar =  200 μm. Box plots of the angle of marker genes show first and third quartile, median is represented by a line, whiskers indicate the minimum and maximum. Each dot represents one embryo.P-values from unpaired two-tailed t-tests are indicated.iPhenotypes of 27 hpf larvae injected with control (mKO2) orrelmRNA. The strength of ventralization was scored. Lateral views with anterior to the left. Scale bar = 200 μm. Source data are provided as a Source Data file. MO sequences are shown in Supplementary Table 1 . LPS (12 ng) from Escherichia coli O111:B4 (L2630; Sigma-Aldrich, St. Louis, MO, USA) was injected at the single-cell stage of the embryos. RNA probe synthesis and whole-mount in situ hybridization RNA probes were generated using gene-specific sequences cloned into multi-cloning sites of pBluescript SK+, pCS2p+, or pCRII-TOPO vectors (Thermo Fisher Scientific, Waltham, MA, USA). Linearized templates were subjected to in vitro transcription with DIG- or FITC-conjugated NTP (Sigma-Aldrich) using T3 (Promega) T7 or SP6 RNA polymerase (Takara), and then purified with RNA Clean & Concentrator Kits (Zymo Research, Irvine, CA, USA). The probe for chordin was preciously described [28] . For rela , the cDNA cloned into the pCR4-TOPO vector was purchased from TransOMIC (Huntsville, AL, USA). The Xho1-digested plasmid was subjected to in vitro transcription using T7 polymerase. 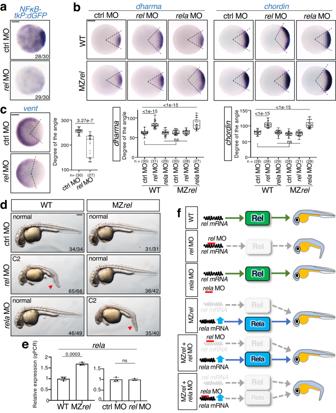Fig. 2: SpecificrelMO reveals that Rel restricts dorsal organizer formation. aRel is a main NFκB acting in early zebrafish embryos. WISH fordGFPin NFκB-tkP:dGFP-transgenic embryos injected with control MO (ctrl MO) orrelMO at dome stage, animal view. Scale bar = 200 μm.b–drelMO leads to expansion of organizer size and dorsal tissue in wild-type (WT) embryos whereasrelacompensates the loss ofrelin MZrelembryos. WISH for (b)dharma,chordin, and (c)vent(ventral marker) in WT and maternal-zygoticrelmutants (MZrel) embryos injected with ctrl MO,relMO orrelaMO at 30% epiboly. Animal views with dorsal to the right. Scale bar = 200 μm. Box plots of the angle of marker genes show first and third quartile, median is represented by a line, whiskers indicate the minimum and maximum. Each dot represents one embryo.P-values from two-tailed one-way ANOVAs with Sidak correction are indicated. ns: not significant (p> 0.05).dRepresentative pictures of 27 hpf WT and MZrellarvae injected with ctrl MO,relMO orrelaMO. The strength of dorsalization was scored. The loss of ventral tail fin is indicated with red arrowheads. Lateral views with anterior to the left. Scale bar = 200 μm.erelais upregulated in MZrelbut notrelmorphants. qPCR analysis for expression ofrelain MZrelorrelmorphants at sphere stage. Normalized values are shown as means ± SEM.n= 3, biologically independent samples.P-values from unpaired two-tailed t-tests are indicated.fModel of the mechanism ofrela-mediated genetic compensation and the specific inhibition byrelMO. Source data are provided as a Source Data file. Primer sequences used for cloning of other probes are shown in Supplementary Table 2 . Whole-mount in situ hybridization was performed according to a standard protocol. Fluorescence in situ hybridization was performed according to a previously described protocol [99] . In brief, embryos were fixed by 4% paraformaldehyde at 4 °C overnight and dehydrated in methanol at −20 °C overnight. Then, embryos were hybridized with FITC- or DIG-labeled RNA probes in Pre-Hyb solution (50% formamide, 5X SSC, 100 μg/ml yeast RNA, 50 μg/ml Heparin, 0.25% tween-20, 0.01 M Citric acid, pH 6.0–6.5) overnight at 68 °C, followed by stringent washes. Embryos were incubated with anti-Fluor-POD or anti-DIG-POD (Roche, Basel, Switzerland) overnight at 4 °C and then incubated with FITC-, Cy3-, or Cy5-tyramide (Akoya Biosciences, Marlborough, MA, USA). 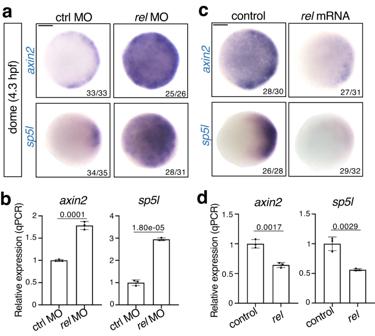Fig. 3: Rel negatively regulates Wnt/β-catenin signaling. Wnt/β-catenin signaling is enhanced byrelknockdown (a,b) and decreased byreloverexpression (c,d) at the dome stage. WISH (a,c) and qPCR analysis (b,d) ofaxin2andsp5lin dome-stage WT embryos injected with ctrl MO,relMO, control (mKO2) orrelmRNA. Inaandc, animal views are shown. Scale bar = 200 μm. Inbandd, normalized values are shown as mean ± SEM.n= 3 biologically independent samples.P-values from unpaired two-tailedt-tests are indicated. Source data are provided as a Source Data file. Images were taken using an M205A stereomicroscope (Leica Microsystems, Wetzlar, Germany) and an FV3000 confocal laser scanning microscope (Evident, Tokyo, Japan). Luciferase assay in zebrafish embryos Frzb-luc plasmid (30 pg) was injected into one-cell-stage zebrafish embryos to detect frzb promoter activity. Fluorescent in situ hybridization (FISH) for luciferase was performed according to a previously described protocol [99] . Images were taken using a M205A stereomicroscope. Genomic DNA isolation and Southern blot analysis The tail fins of adult transgenic fish were amputated using a razor and transferred to a lysis buffer containing 0.1 μg/μl Proteinase K (ProK). The samples were incubated overnight at 55 °C, followed by standard ethanol precipitation. Purified genomic DNA samples were digested with EcoRI, which cuts the plasmid reporter. Southern blot hybridization was performed using a digoxigenin (Roche, Basel, Switzerland)-labeled probe and standard methods. Quantitative PCR Zebrafish embryos were randomly collected. Total RNA content from 25 embryos was purified using TRIzol reagent (Invitrogen), and cDNA was synthesized using ReverTra Ace qPCR RT Master Mix (Toyobo, Osaka, Japan). Quantitative PCR (qPCR) was performed on an Mx3000P QPCR system (Agilent Technologies) with THUNDERBIRD SYBR qPCR Mix (Toyobo), and qPCR was performed in triplicate. The levels of actb1 , ef1α, and rpl13 were used as a loading control. qPCR cycling conditions were as follows: 95 °C for 1 min, [95 °C for 10 s, and 60 °C for 30 s] (45 cycles), followed by dissociation curve analysis. The primer list is shown in Supplementary Table 1 . Cell culture and transfection HEK293 cells (#CRL-1573™, ATCC) were grown in Dulbecco’s modified Eagle’s medium (DMEM) supplemented with 10% foetal bovine serum (FBS) and 100 U/ml penicillin-streptomycin (Nacalai Tesque, Kyoto, Japan). Cells were transfected with expression plasmids encoding zebrafish Rel, mouse c-Rel, and the NFκB signaling activators TAB1 and TAK1 [100] and reporter plasmids using polyethyleneimine MW 25000 (Polysciences, Warrington, PA, USA). 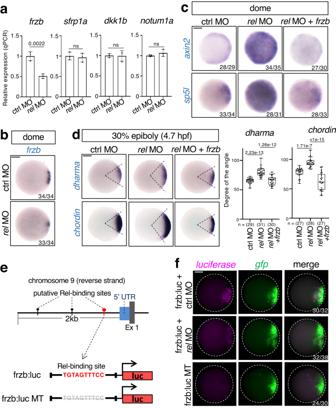Fig. 4: Rel directly activates a secreted Wnt antagonist Frzb to restrict Wnt/β-catenin-mediated dorsal organizer formation. a,bRel positively regulatesfrzbexpression.aqPCR analysis for expression of Wnt antagonists (frzb,sfrp1a,dkk1bandnotum1a) in dome stage embryos injected with ctrl MO orrelMO. Normalized values are shown as means ± SEM.n= 3, biologically independent samples.P-values from unpaired two-tailed t-tests are indicated.bWISH forfrzbin dome stage embryos injected with ctrl MO orrelMO, animal view.c,dRel inhibits Wnt/β-catenin signaling through Frzb. WISH for (c) Wnt targetsaxin2andsp5l; (d)dharmaandchordinin embryos injected with ctrl MO,relMO orrelMO withfrzbmRNA at indicated stage, animal view. Box plots of the angle of marker genes show first and third quartile, median is represented by a line, whiskers indicate the minimum and maximum. Each dot represents one embryo.P-values from two-tailed one-way ANOVAs with Sidak correction are indicated.e,fRel activates promoter offrzb.eTop panel shows the schematic diagram of the upstream region of zebrafishfrzbgene. The NFκB-binding element possessing the strongest potential to bind to Rel homodimer is marked with red “pin” while others are marked by black “pins”. Gray and blue boxes indicate Exons and UTRs, respectively. Bottom panel shows the schematic diagrams of the reporter constructs, frzb:luc and frzb:luc MT.fFISH forluciferase(magenta) andgfp(green) in dome-stage embryos injected with pDha-GFP and frzb:luc or frzb:luc MT, with MOs as indicated, animal view. Scale bar = 200 μm. Source data are provided as a Source Data file. Chemical treatment TAK-242 (243984-11-4; Cayman Chemical, Ann Arbor, MI, USA) was dissolved in dimethyl sulfoxide (DMSO) at 10 mg/ml and stored at −30 °C. TAK-242 (40 μM) was treated from 3 hpf. To observe the phenotype at 27 hpf, embryos were washed thrice with egg water at 4.7 hpf to remove TAK-242. Statistics and reproducibility Statistical analyses were performed using GraphPad Prism software v8.0.1 (GraphPad Software, Boston, MA, USA). The statistical significance of differences between groups in all datasets was calculated using a two-tailed unpaired t-test or one-way analysis of variance. P -values ≤ 0.05 were considered statistically significant. Figures of representative images or plots were reproduced in at least two (Figs. 4 b–d, f, 5 a–f, and 6a–h and Supplementary Figs. 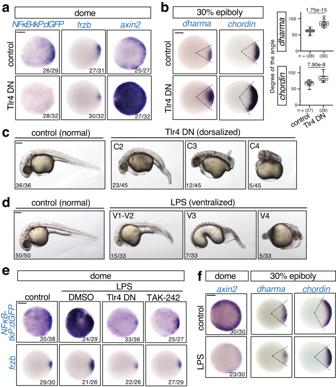Fig. 5: Tlr4 activates NFκB to stimulatefrzb-mediated restriction of dorsal organizer formation. a–cInhibition of Tlr4 reducesfrzbexpression and enhances Wnt/β-catenin signaling and dorsal organizer formation. Embryos were injected with mKO2 (control) or Tlr4 DN mRNA. WISH for (a)dGFPin NFκB-tkP:dGFP-transgenic;frzbandaxin2in WT, (b)dharmaandchordinin WT embryos at the indicated stage. Animal views. Box plots of the angle of marker genes show first and third quartile, median is represented by a line, whiskers indicate the minimum and maximum. Each dot represents one embryo.P-values from unpaired two-tailed t-tests are indicated.cRepresentative pictures of 27 hpf larvae, lateral views with anterior to the left. The strength of dorsalization was scored.d–fForced activation of Tlr4 by injection of lipopolysaccharide (LPS) activates NFκB signaling and inhibits dorsal organizer formation.dPhenotypes of 27 hpf larvae injected with LPS, uninjected as control. The strength of ventralization was scored. Lateral views with anterior to the left.eEmbryos were injected with LPS and treated with DMSO or TAK-242 or co-injected with Tlr4 DN, uninjected as control. DMSO and TAK-242 were treated from 3 hpf to dome stage. WISH fordGFPin NFκB-tkP:dGFP-transgenic;frzbin WT embryos at dome stage.fWISH foraxin2,dharmaandchordinin embryos injected with LPS, uninjected as control. Animal views. Scale bar = 200 μm. Source data are provided as a Source Data file. 1a –d, 2d , 2f , 3c , d, 4a –e, 5a , b, and 6a ), or three or more (Figs. 1 a–i, 2 a–e, 3 a–d and 4a and Supplementary Figs. 2b , c, e , 2g , i , 3a , b, 5c –f, and 6b ) independent experiments. No statistical method was used to predetermine the sample size. No data were excluded from the analyses. Animals were randomly assigned to each experimental group. The Investigators were not blinded to allocation during experiments and outcome assessment. 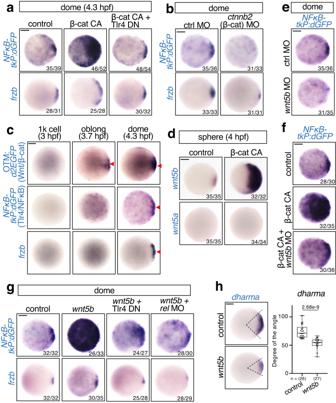Fig. 6: β-catenin stimulates Wnt5b-mediated Tlr4/NFκB activation. a,bβ-catenin activates NFκB via Tlr4.aEmbryos were injected with control (mKO2) or constitutively active β-catenin mutant (β-cat CA) mRNA, with or without Tlr4 DN mRNA.bEmbryos were injected with control orctnnb2(zebrafish β-catenin) MO. WISH fordGFPin NFκB-tkP:dGFP-transgenic;frzbin WT embryos at the dome stage, animal view. Scale bar = 200 μm.cNFκB is activated following Wnt/β-catenin activation in the developing dorsal organizer. WISH fordGFPin OTM:d2EGFP and NFκB-tkP:dGFP-transgenic embryos andfrzbin WT embryos at the indicated stage. ThedGFP-expressing andfrzb-expressing dorsal regions are indicated by red arrowheads. Scale bar = 200 μm.dβ-catenin activateswnt5bexpression in early embryos. Embryos were injected with control (mKO2) or constitutively active β-catenin mutant (β-catCA) mRNA. WISH forwnt5aandwnt5bat the sphere stage, animal view. Scale bar = 200 μm.e,fWnt/β-catenin signaling activates NFκB via Wnt5b.eEmbryos were injected with ctrl orwnt5bMO.fEmbryos were injected with control (mKO2) or constitutively active β-catenin mutant (β-cat CA) mRNA, with or withoutwnt5bMO. WISH fordGFPin NFκB-tkP:dGFP-transgenic embryos at the dome stage, animal view. Scale bar = 200 μm.g,hWnt5b activatesfrzbexpression through Tlr4/Rel.gEmbryos were injected with control (mKO2) orwnt5bmRNA, and co-injected with Tlr4 DN mRNA orrelMO. WISH fordGFPin NFκB-tkP:dGFP-transgenic,frzbin WT embryos at the dome stage, animal view. Scale bar = 200 μm.hWISH fordharmain WT embryos injected with control (mKO2) orwnt5bmRNA at 30% epiboly stage. Scale bar = 200 μm. Box plots of the angle of marker gene show first and third quartile, median is represented by a line, whiskers indicate the minimum and maximum. Each dot represents one embryo.P-values for unpaired two-tailed t-tests are indicated. Source data are provided as a Source Data file. 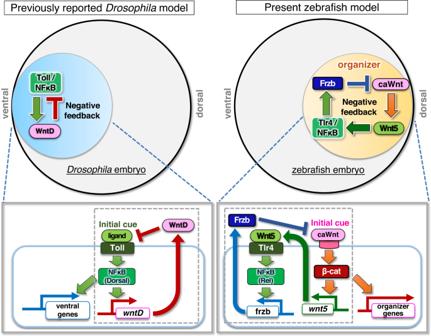Fig. 7: Negative feedback loop between canonical/non-canonical Wnts and Tlr4/NFκB determines the precise size of zebrafish dorsal organizer. Model of the role of Tlr/NFκB signaling in the initiation of embryonic DV axis formation. InDrosophila, Wnt-mediated negative feedback regulation of Toll/NFκB signaling determines the embryonic DV pattern. In zebrafish, negative feedback regulation between canonical Wnt (caWnt), non-canonical Wnt (Wnt5b), and Tlr4/NFκB generates the precise size of the dorsal organizer and the consequent DV pattern. Reporting summary Further information on research design is available in the Nature Portfolio Reporting Summary linked to this article.